Monitoring and robust induction of nephrogenic intermediate mesoderm from human pluripotent stem cells A method for stimulating the differentiation of human pluripotent stem cells into kidney lineages remains to be developed. Most cells in kidney are derived from an embryonic germ layer known as intermediate mesoderm. Here we show the establishment of an efficient system of homologous recombination in human pluripotent stem cells by means of bacterial artificial chromosome-based vectors and single-nucleotide polymorphism array-based detection. This system allowed us to generate human-induced pluripotent stem cell lines containing green fluorescence protein knocked into OSR1 , a specific intermediate mesoderm marker. We have also established a robust induction protocol for intermediate mesoderm, which produces up to 90% OSR1 + cells. These human intermediate mesoderm cells can differentiate into multiple cell types of intermediate mesoderm-derived organs in vitro and in vivo , thereby supplying a useful system to elucidate the mechanisms of intermediate mesoderm development and potentially providing a cell source for regenerative therapies of the kidney. The kidneys have highly differentiated and complicated structures, and have pivotal roles in many physiological processes, such as the regulation of fluid and electrolyte balance, body fluid osmolality, the acid–base balance, the excretion of metabolic waste products and foreign chemicals, and the production of hormones controlling blood pressure and erythropoiesis. Once damaged, kidneys rarely recover their functions. The renal tubules can regenerate to some extent in the case of acute tubular necrosis, but kidneys generally do not regenerate in patients with chronic kidney diseases [1] . This failure to fully regenerate cause the progression to end-stage renal insufficiency. An increasing number of patients suffer from end-stage renal disease [2] , and there is a shortage of donor kidneys for transplantation around the world. Most of the patients must undergo dialysis therapy for the remainder of their lives, which causes both medical and medico-economical problems. To overcome this problem, kidney regeneration using embryonic stem cells (ESCs) [3] , [4] , [5] or induced pluripotent stem cells (iPSCs) [6] , [7] , [8] , which have an unlimited self-renewal capability and the potential to differentiate into any cell type in the body, is a valuable alternative. The induction of renal lineage cells has been performed using mouse ESCs, while a method to induce the differentiation of human pluripotent stem cells (hPSCs) into the renal lineage has not yet been fully established [9] , [10] , [11] , [12] , [13] , [14] , [15] . Kidneys are derived from the intermediate mesoderm (IM), and Odd-skipped related 1 ( Osr1 ) is one of the earliest markers specific for IM, although the expression also extends into the lateral plate mesoderm at early stages in mouse, chick and fish embryos [16] , [17] , [18] . The differentiation of PSCs into OSR1- expressing IM cells is the first step toward the induction of renal lineage cells. In our present study, we initially constructed bacterial artificial chromosome (BAC)-based vectors and transduced them into hiPSCs to obtain reporter hiPSC lines for an IM marker gene, OSR1 , by homologous recombination. By using these lines and conducting combinational treatments with growth factors, we have established a robust induction protocol for IM, which produces up to 90% OSR1 + cells. We have also confirmed that these hiPSC-derived IM cells have similar developmental potential to those found in embryos, and that they can differentiate into multiple cell types included in IM-derivative organs, such as the kidneys, gonads and adrenal cortex Generation of OSR1-GFP knock-in hiPSC lines We initially constructed a conventional targeting vector with 5 and 3 kb homologous arms to generate OSR1-GFP reporter hiPSC lines to monitor their differentiation into IM, but did not obtain a homologous recombinant in the more than 1,300 drug-resistant clones we examined (data not shown). Therefore, we adopted a strategy using BAC-based vectors shown in Fig. 1a to establish OSR1-GFP knock-in lines. A previously derived hiPSC line, 201B7 ( [7] ), was used as a parental line. Notably, four clones, 3D36, 3D45, 3F3 and 3I49, were selected as candidate lines with homologous recombination from ~130 drug-resistant clones by using a Taqman quantitative PCR (qPCR) analysis to detect the loss of an OSR1 -coding region, which was replaced by a GFP-Neo cassette ( Fig. 1b ). 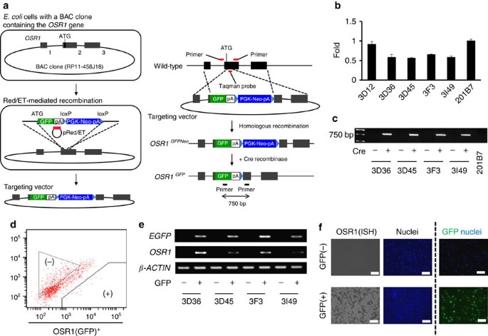Figure 1: Generation of OSR1-GFP knock-in hiPSC lines. (a) A schematic representation of the targeting strategy using BAC-based vectors to produce OSR1-GFP knock-in hiPSC lines. A part of theOSR1cording region was replaced by EGFP and PGK-Neo cassettes. The black boxes represent three exons of theOSR1gene. (b) The Taqman qPCR analysis of genomic DNA from the drug-resistant lines and the parental line (201B7). Note that a value of 1 indicates two intactOSR1loci, while 0.5 suggests one intact and one targeted locus. 3D12 is a drug-resistant clone without homologous recombination. The Taqman probe and the primer pair indicated ina(red bars) was used. The data from three independent experiments are presented as the mean±s.d. (n=3). (c) Genomic PCR was used to confirm the removal of the Neo cassette by Cre recombination. The primer pair indicated ina(black bars) was used. (d) The flow cytometric analysis of OSR1 (GFP)+cells on culture day 16 of spontaneously differentiating EB without any inducing factors. (e) The results of the RT–PCR analyses of the GFP+and GFP−populations isolated on day 16 that were shown ind. (f)In situhybridization (ISH) analysis using specific probes againstOSR1and immnostaining using antibodies against GFP on the GFP+and GFP−cells on culture day 16. Scale bars, 100 μm. Figure 1: Generation of OSR1-GFP knock-in hiPSC lines. ( a ) A schematic representation of the targeting strategy using BAC-based vectors to produce OSR1-GFP knock-in hiPSC lines. A part of the OSR1 cording region was replaced by EGFP and PGK-Neo cassettes. The black boxes represent three exons of the OSR1 gene. ( b ) The Taqman qPCR analysis of genomic DNA from the drug-resistant lines and the parental line (201B7). Note that a value of 1 indicates two intact OSR1 loci, while 0.5 suggests one intact and one targeted locus. 3D12 is a drug-resistant clone without homologous recombination. The Taqman probe and the primer pair indicated in a (red bars) was used. The data from three independent experiments are presented as the mean±s.d. ( n =3). ( c ) Genomic PCR was used to confirm the removal of the Neo cassette by Cre recombination. The primer pair indicated in a (black bars) was used. ( d ) The flow cytometric analysis of OSR1 (GFP) + cells on culture day 16 of spontaneously differentiating EB without any inducing factors. ( e ) The results of the RT–PCR analyses of the GFP + and GFP − populations isolated on day 16 that were shown in d . ( f ) In situ hybridization (ISH) analysis using specific probes against OSR1 and immnostaining using antibodies against GFP on the GFP + and GFP − cells on culture day 16. Scale bars, 100 μm. Full size image A single-nucleotide polymorphism (SNP) array analysis was utilized to examine the copy number of the OSR1 gene, and this indicated that the four clones had two loci, one of which was intact except for the GFP-Neo inserted region, whereas non-candidate clones, such as 3D12, showed three copies ( Fig. 2a ). Thus, the SNP array analysis confirmed the generation of four knock-in lines. This analysis also showed no other apparent genetic alterations, except that clone 3I49 has a copy number variation in chromosome 9 ( Fig. 2b , arrows). The G-banding analysis of the four clones showed a normal karyotype ( Supplementary Fig. S1 ). The Neo cassette was excised at the flanking loxP sites by transient expression of Cre-recombinase, and the elimination was confirmed by genomic PCR ( Fig. 1c ). 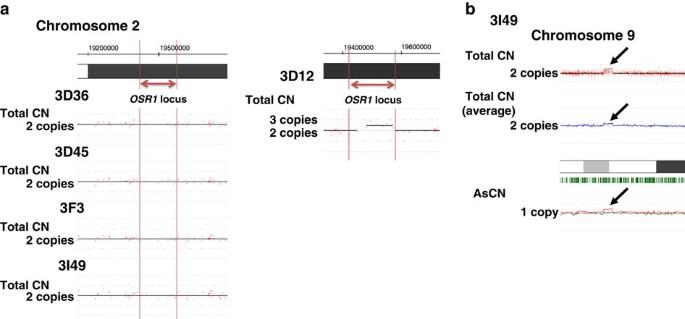Figure 2: SNP array analysis of OSR1-GFP reporter hiPSC lines. (a) The copy number (CN) ofOSR1gene loci was analysed by the number of SNPs in the five reporter hiPSC lines; 3D36, 3D45, 3F3, 3I49 and 3D12. Genomic DNA from the parental line (201B7) and the five reporter lines was analysed by GeneChip Mapping 250K NSP arrays. The genomic CNs, including AsCNs, were calculated using the CNAG/AsCNAR software program. On each panel, the red dots andyaxis represent the signal intensity of each SNP probe, and CNs (black lines) were detected using a hidden Markov model-based algorithm implemented in the CNAG/AsCNAR software program. CNs were normalized to the samples of 201B7. Note that 3D36, 3D45, 3F3 and 3I49 (CN=2) are knock-in lines with homologous recombination, whereas 3D12 (CN=3) is a drug-resistant transgenic line without homologous recombination. (b) The copy number variation in chromosome 9 (black arrows) of a reporter hiPSC line, 3I49. The blue line in the upper middle represents the averaged total CNs, and heterozygous SNP calls are marked with the green bars beneath the chromosomes shown as white, grey and black boxes in the bottom middle. The red and green lines in the bottom represent the moving average of AsCNs. Figure 2: SNP array analysis of OSR1-GFP reporter hiPSC lines. ( a ) The copy number (CN) of OSR1 gene loci was analysed by the number of SNPs in the five reporter hiPSC lines; 3D36, 3D45, 3F3, 3I49 and 3D12. Genomic DNA from the parental line (201B7) and the five reporter lines was analysed by GeneChip Mapping 250K NSP arrays. The genomic CNs, including AsCNs, were calculated using the CNAG/AsCNAR software program. On each panel, the red dots and y axis represent the signal intensity of each SNP probe, and CNs (black lines) were detected using a hidden Markov model-based algorithm implemented in the CNAG/AsCNAR software program. CNs were normalized to the samples of 201B7. Note that 3D36, 3D45, 3F3 and 3I49 (CN=2) are knock-in lines with homologous recombination, whereas 3D12 (CN=3) is a drug-resistant transgenic line without homologous recombination. ( b ) The copy number variation in chromosome 9 (black arrows) of a reporter hiPSC line, 3I49. The blue line in the upper middle represents the averaged total CNs, and heterozygous SNP calls are marked with the green bars beneath the chromosomes shown as white, grey and black boxes in the bottom middle. The red and green lines in the bottom represent the moving average of AsCNs. Full size image Next, OSR1 + cells were induced from the four lines by spontaneous differentiation using embryoid body (EB) formation without any inducing factors, and then were isolated by flow cytometry for RT–PCR (PCR with reverse transcription) analyses, which showed that only GFP + cells expressed OSR1 in all four lines ( Fig. 1d ). Moreover, in situ hybridization analyses of clone 3D45 using OSR1 probes showed that almost all GFP + cells expressed OSR1 transcripts, whereas the GFP − cells did not, thereby confirming the correlation between GFP and OSR1 expression ( Fig. 1f ). These results suggested that OSR1-GFP knock-in hiPSC lines had been efficiently generated using BAC-based vectors and the detection systems for homologous recombinants using the Taqman qPCR and SNP array analyses, and that these reporter lines can be used for monitoring OSR1 + cells differentiated from hiPSCs. Establishment of robust induction methods of IM cells To establish protocols for the differentiation of IM from hPSCs, we examined the effects of ~40 different growth factors on hESC differentiation and found that bone morphogenetic protein (BMP) 7 was the most potent inducer of OSR1 expression ( Supplementary Fig. S2 ). We next examined the mesendoderm (ME) induction step before BMP7 treatment to increase the efficiency of IM differentiation. We used 100 ng ml −1 of activin A and Wnt3a to differentiate hPSCs into ME cells, as the factors had previously been shown to induce the differentiation from PSCs [19] , [20] . As expected, the treatment induced EBs from an OSR1 reporter hiPSC line, 3D45, to express ME markers, BRACHYURY , GSC and MIXL1 , but not ectodermal ( SOX1 and PAX6 ) or endodermal ( SOX17 and FOXA2 ) marker expression ( Supplementary Fig. S3a ). Adding either or both SB431542 (an inhibitor of TGFβ receptor kinase) and Frizzled-Fc chimeric protein (an antagonist of the Wnt pathway) decreased the expression of BRACHYURY , thus confirming the involvement of activin A and Wnt signalling in the ME differentiation ( Supplementary Fig. S3b ). For IM induction, we confirmed that the combination of the ME induction step (Stage 1) and subsequent BMP7 treatment (Stage 2) produced higher OSR1 expression than BMP7 treatment alone, and also found that the addition of Wnt3a to BMP7 in Stage 2 led to even higher expression than BMP7 alone ( Fig. 3a ). The suppression of OSR1 expression by adding either or both Noggin (an antagonist of BMPs) and Frizzled-Fc chimeric proteins suggested that BMP7 and Wnt3a signals are essential for the induction of OSR1 -expressing cells ( Fig. 3c ). 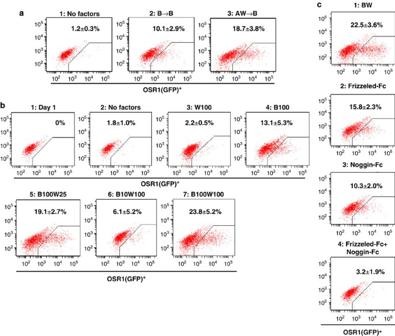Figure 3: Differentiation of hiPSCs into the intermediate mesoderm. (a) Flow cytometric analyses of OSR1(GFP)+cell differentiation on culture day 11. 1: no factors; 2: 100 ng ml−1BMP7; 3: Stage 1, 100 ng ml−1activin A+100 ng ml−1Wnt3a, Stage 2, 100 ng ml−1BMP7. (b) The differentiation of OSR1(GFP)+cells on culture day 11, analysed by flow cytometry. 1: on day 1 before treatments; 2: no factors; 3–7: Stage 1, 100 ng ml−1activin A+100 ng ml−1Wnt3a. The treatments at stage 2 are as follows, 3: 100 ng ml−1Wnt3a; 4: 100 ng ml−1BMP7; 5: 100 ng ml−1BMP7+25 ng ml−1Wnt3a; 6: 10 ng ml−1BMP7+100 ng ml−1Wnt3a; 7: 100 ng ml−1BMP7+100 ng ml−1Wnt3a. (c) The suppression of the induction efficiency of OSR1(GFP)+cells on culture day 11 by adding Frizzled- and/or Noggin-Fc chimeric proteins to the treatment with 100 ng ml−1BMP7+100 ng ml−1Wnt3a at Stage 2. The treatment at Stage 1 is 100 ng ml−1activin A+100 ng ml−1Wnt3a in all experiments. 1: without Frizzled- or Noggin-Fc; 2: 1 mg ml−1Frizzled-Fc; 3: 1 mg ml−1Noggin-Fc; 4: 1 mg ml−1Frizzled-Fc+1 mg ml−1Noggin-Fc. The data from three independent experiments are presented as the means±s.d. (n=3). Figure 3: Differentiation of hiPSCs into the intermediate mesoderm. ( a ) Flow cytometric analyses of OSR1(GFP) + cell differentiation on culture day 11. 1: no factors; 2: 100 ng ml −1 BMP7; 3: Stage 1, 100 ng ml −1 activin A+100 ng ml −1 Wnt3a, Stage 2, 100 ng ml −1 BMP7. ( b ) The differentiation of OSR1(GFP) + cells on culture day 11, analysed by flow cytometry. 1: on day 1 before treatments; 2: no factors; 3–7: Stage 1, 100 ng ml −1 activin A+100 ng ml −1 Wnt3a. The treatments at stage 2 are as follows, 3: 100 ng ml −1 Wnt3a; 4: 100 ng ml −1 BMP7; 5: 100 ng ml −1 BMP7+25 ng ml −1 Wnt3a; 6: 10 ng ml −1 BMP7+100 ng ml −1 Wnt3a; 7: 100 ng ml −1 BMP7+100 ng ml −1 Wnt3a. ( c ) The suppression of the induction efficiency of OSR1(GFP) + cells on culture day 11 by adding Frizzled- and/or Noggin-Fc chimeric proteins to the treatment with 100 ng ml −1 BMP7+100 ng ml −1 Wnt3a at Stage 2. The treatment at Stage 1 is 100 ng ml −1 activin A+100 ng ml −1 Wnt3a in all experiments. 1: without Frizzled- or Noggin-Fc; 2: 1 mg ml −1 Frizzled-Fc; 3: 1 mg ml −1 Noggin-Fc; 4: 1 mg ml −1 Frizzled-Fc+1 mg ml −1 Noggin-Fc. The data from three independent experiments are presented as the means±s.d. ( n =3). Full size image We next analysed the temporal expression pattern of OSR1 by qRT–PCR and found a gradual increase, with a peak at culture day 19 ( Fig. 4a ). Flow cytometric analyses using 3D45 showed the induction rate of OSR1 + cells to increase up to more than 40% on day 19, which was consistent with the qRT–PCR results ( Fig. 4b ). 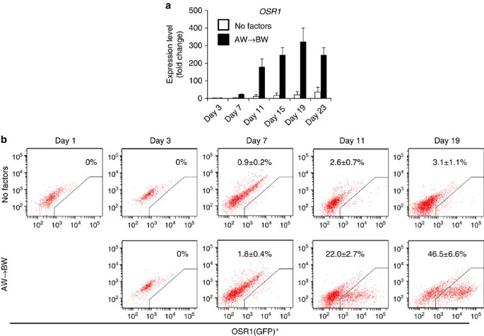Figure 4: Differentiation pattern of OSR1+cells using the EB-based induction method. (a) The time course analysis ofOSR1expression. Each value was normalized to the samples on day 1 before treatments. White bars: no factors; black bars (AW→BW): Stage 1, 100 ng ml−1activin A+100 ng ml−1Wnt3a; Stage 2, 100 ng ml−1BMP7+100 ng ml−1Wnt3a. Note that theOSR1expression on day 3 is so low that the histogram bars are at the baseline. (b) The differentiation course of OSR1(GFP)+cells was analysed by flow cytometry. The data from three independent experiments are presented as the means±s.d. (n=3) inaandb. Figure 4: Differentiation pattern of OSR1 + cells using the EB-based induction method. ( a ) The time course analysis of OSR1 expression. Each value was normalized to the samples on day 1 before treatments. White bars: no factors; black bars (AW→BW): Stage 1, 100 ng ml −1 activin A+100 ng ml −1 Wnt3a; Stage 2, 100 ng ml −1 BMP7+100 ng ml −1 Wnt3a. Note that the OSR1 expression on day 3 is so low that the histogram bars are at the baseline. ( b ) The differentiation course of OSR1(GFP) + cells was analysed by flow cytometry. The data from three independent experiments are presented as the means±s.d. ( n =3) in a and b . Full size image We next examined the substitution of CHIR99021, a specific inhibitor of glycogen synthase kinase (GSK) 3β that activates canonical Wnt signalling, for Wnt3a in the differentiation protocol ( Supplementary Fig. S4 ). OSR1 + cells were more efficiently induced with 1 μM CHIR99021 than with 100 ng ml −1 Wnt3a. In addition, 6-bromoindirubin-3′-oxime, another GSK3β inhibitor, showed similar effects on the differentiation (data not shown). These results suggest that the Wnt3a protein can be replaced by synthetic GSK3β inhibitors, and that the canonical Wnt pathway is involved in IM differentiation. The complexity of EBs and the contamination of feeder cells make it difficult to analyse the molecular signals and cellular interactions involved in differentiation processes. We therefore tested the same inducing factors in two-dimensional monolayer culture without feeder layers (colony method, Supplementary Fig. S5 ). OSR1 + cells were produced under these conditions with either of Wnt3a or CHIR99021, although the induction rate (about 15% on day 11) was lower than that with EB-based three-dimensional culture (EB method, Fig. 4 ). To improve the induction efficiency, we created a novel two-dimensional culture system, in which hPSCs were gently dissociated into single cells with Accutase, and the addition of a ROCK inhibitor (Y27,632) increased the survival and differentiation of single hPSCs (single-cell method). Notably, the induction rate of OSR1 + cells at culture day 11 increased up to 90% when 3 μM CHIR99021 was used with activin A at Stage 1 and BMP7 at Stage 2 ( Fig. 5a and Supplementary Fig. S6a ). These results were confirmed by qRT–PCR analysis of OSR1 expression and in situ hybridization using OSR1 probes ( Fig. 5b and Supplementary Fig. S6b ). The single-cell method more efficiently induced OSR1 + cells and produced more than 10-fold higher OSR1 expression than the EB or colony methods ( Fig. 5c and Supplementary Fig. S7a ), which was consistent with the flow cytometric findings that the protocol more frequently generated cells expressing high levels of OSR1 than other methods ( Supplementary Fig. S7b ). 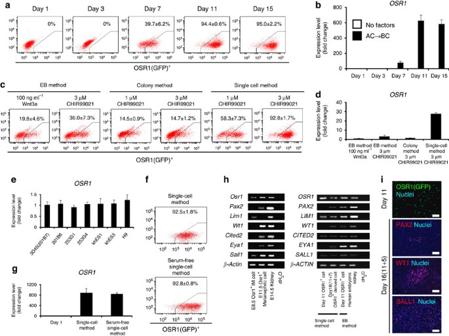Figure 5: Establishing methods for differentiating hPSCs into OSR1+cells. (a) Temporal differentiation pattern of OSR1+cells using the single-cell method. (b) Time course analysis ofOSR1expression in the differentiation culture with the single-cell method. Each value was normalized to the samples on day 1 before treatments. Black bars (AC→BC): Stage 1, 100 ng ml−1activin A+3 μM CHIR99021; Stage 2, 100 ng ml−1BMP7+3 μM CHIR99021. Note that theOSR1expression of samples on culture days 1 and 3 and without factors is so low that histogram bars are at the baseline. (c) The induction rate of OSR1+cells on day 11 obtained using the three induction protocols; EB-based three-dimensional culture (EB method), feeder-free monolayer culture (colony method), and feeder-free monolayer culture with single-cell dissociation (single-cell method). (d) TheOSR1expression in the 3D45 clone resulting from the three induction methods. (e) A comparison of theOSR1expression on day 11 in multiple hiPSC/ESC lines treated with the single-cell method. Samples of 3D45 were used as controls to normalize the data. (f) The differentiation of OSR1+cells on day 11 using the serum-free single-cell method. (g) TheOSR1expression in the serum-free single-cell method. (h) RT–PCR analyses of marker gene expression for IM or kidney lineage in Osr1+cells isolated from E8.5 and E11.5 mouse embryos, isolated OSR1+cells differentiated from 3D45 on day 11 using two induction protocols (EB and single-cell methods), and the differentiated cells on day 18 (after an additional 7-day culture of the day 11 isolated OSR1+cells generated with the single-cell method). (i) Immunostaining of isolated OSR1+cells on day 11 generated with the single-cell method, and the differentiated cells on day 16 (after an additional 5-day culture of the day 11 isolated OSR1+cells) using antibodies against GFP and other IM markers. The cells were isolated by flow cytometry and then spun down onto slides. The data from three independent experiments are presented as the means±s.d. (n=3) ina–g. Scale bars, 100 μm. Figure 5: Establishing methods for differentiating hPSCs into OSR1 + cells. ( a ) Temporal differentiation pattern of OSR1 + cells using the single-cell method. ( b ) Time course analysis of OSR1 expression in the differentiation culture with the single-cell method. Each value was normalized to the samples on day 1 before treatments. Black bars (AC→BC): Stage 1, 100 ng ml −1 activin A+3 μM CHIR99021; Stage 2, 100 ng ml −1 BMP7+3 μM CHIR99021. Note that the OSR1 expression of samples on culture days 1 and 3 and without factors is so low that histogram bars are at the baseline. ( c ) The induction rate of OSR1 + cells on day 11 obtained using the three induction protocols; EB-based three-dimensional culture (EB method), feeder-free monolayer culture (colony method), and feeder-free monolayer culture with single-cell dissociation (single-cell method). ( d ) The OSR1 expression in the 3D45 clone resulting from the three induction methods. ( e ) A comparison of the OSR1 expression on day 11 in multiple hiPSC/ESC lines treated with the single-cell method. Samples of 3D45 were used as controls to normalize the data. ( f ) The differentiation of OSR1 + cells on day 11 using the serum-free single-cell method. ( g ) The OSR1 expression in the serum-free single-cell method. ( h ) RT–PCR analyses of marker gene expression for IM or kidney lineage in Osr1 + cells isolated from E8.5 and E11.5 mouse embryos, isolated OSR1 + cells differentiated from 3D45 on day 11 using two induction protocols (EB and single-cell methods), and the differentiated cells on day 18 (after an additional 7-day culture of the day 11 isolated OSR1 + cells generated with the single-cell method). ( i ) Immunostaining of isolated OSR1 + cells on day 11 generated with the single-cell method, and the differentiated cells on day 16 (after an additional 5-day culture of the day 11 isolated OSR1 + cells) using antibodies against GFP and other IM markers. The cells were isolated by flow cytometry and then spun down onto slides. The data from three independent experiments are presented as the means±s.d. ( n =3) in a – g . Scale bars, 100 μm. Full size image Different hESC lines have been shown to vary in their differentiation potential [21] . The induction protocols for IM cells was tested on three additional hiPSC lines, 201B6 ( [7] ), 253G1 and 253G4 ( [22] ), and three hESC lines, H9 ( [5] ), khES1 and khES3 ( [23] ) ( Fig. 5e and Supplementary Fig. S8 ). Importantly, the single-cell method induced similar expression levels of OSR1 from all the hPSC lines examined, whereas the EB method was not applicable for one of the hiPSC lines, 253G4. To establish a well-defined differentiation method of PSCs would provide an excellent system for studying the molecular mechanisms underlying differentiation. We therefore devised a serum-free differentiation method by replacing both fetal bovine serum (FBS) used in Stage 1 and knockout serum replacement (KSR) in Stage 2 of the single-cell method with B27 supplement. The induction efficiency of OSR1 + cells in the refined protocol (serum-free single-cell method) was about 90% and comparable to the original single-cell method ( Fig. 5f ). The OSR1 + cells that were differentiated using the single-cell method and isolated on culture day 11 expressed some of the PAX2 , LIM1 , WT1 , CITED2 , EYA1 and SALL1 genes, which are known to be expressed in cells of IM or kidney lineage [10] , and the cells expressed all of the markers after an additional 5–7 days of culture with 100 ng ml −1 BMP7 and 100 ng ml −1 Wnt3a or 1–3 μM CHIR99021 ( Fig. 5h ). The gene expression patterns of the OSR1 + cells isolated on day 11 that were generated using the single-cell method and the cells on day 18 (11+7) were similar to that of embryonic day (E) 8.5 Osr1 + IM and E11.5 Osr1 + metanephric cells obtained from Osr1-GFP knock-in mice [18] , respectively ( Fig. 5h ). Some OSR1 + cells were positive for PAX2, WT1 or SALL1 by immunostaining, which was similar to the findings observed in the IM cells of mouse embryos ( Fig. 5i and Supplementary Fig. S9 ). Although the weak expression of a hematopoietic lineage marker, CD41 , was detected ( Supplementary Fig. S10 ), these results suggested that the novel monolayer culture with single-cell dissociation can efficiently generate OSR1 + cells, and that most of these cells might therefore represent IM. We next examined the applicability of our induction protocols to mouse PSC (mPSC) lines using two iPSC lines, 492B-4 ( [24] ) and 20D-17 ( [25] ), and two ESC lines, D3 and J1 ( Fig. 6 ). In contrast to hPSCs, the EB method did not significantly stimulate the Osr1 expression in any of the four mouse lines. As retinoic acid (RA) was previously used for the renal lineage differentiation of mouse ESCs [10] , we examined the effect of adding RA to the differentiation culture and observed the enhancement of Osr1 expression. However, adding RA to the hPSC differentiation culture did not show any advantageous effects on the IM induction ( Supplementary Fig. S11 ). These results suggest that our differentiation protocols for generating IM cells can be applicable to multiple hPSC lines and that the addition of RA enhances the IM induction from mPSCs. 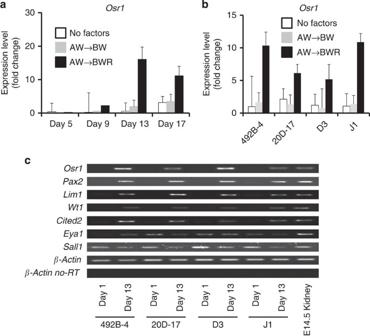Figure 6: The differentiation of multiple miPSC/ESC lines into IM cells. (a) The temporary expression pattern ofOsr1in differentiation culture from a miPSC line, 492B-4. Samples before treatments on day 1 were used as a control. White bars: no factors; grey bars (AW→BW): Stage 1, 100 ng ml−1activin A+100 ng ml−1Wnt3a, Stage 2, 100 ng ml−1BMP7+100 ng ml−1Wnt3a; black bars (AW→BWR): Stage 1, 100 ng ml−1activin A+100 ng ml−1Wnt3a, Stage 2, 100 ng ml−1BMP7+100 ng ml−1Wnt3a+0.1 mM RA. (b) A comparison of theOsr1expression on day 13 of differentiation culture from two miPSC lines (492B-4 and 20D-17) and two mESC lines (D3 and J1). Samples from 492B-4 iPSCs on day 13 were used as a control to normalize data. (c) The expression of IM marker genes analysed by RT–PCR is shown. The data from three independent experiments are presented as the means±s.d. (n=3) inaandb. For mPSCs, we generated EBs without any inducing factors, and then the same two-step treatment was employed as used for hPSCs. Figure 6: The differentiation of multiple miPSC/ESC lines into IM cells. ( a ) The temporary expression pattern of Osr1 in differentiation culture from a miPSC line, 492B-4. Samples before treatments on day 1 were used as a control. White bars: no factors; grey bars (AW→BW): Stage 1, 100 ng ml −1 activin A+100 ng ml −1 Wnt3a, Stage 2, 100 ng ml −1 BMP7+100 ng ml −1 Wnt3a; black bars (AW→BWR): Stage 1, 100 ng ml −1 activin A+100 ng ml −1 Wnt3a, Stage 2, 100 ng ml −1 BMP7+100 ng ml −1 Wnt3a+0.1 mM RA. ( b ) A comparison of the Osr1 expression on day 13 of differentiation culture from two miPSC lines (492B-4 and 20D-17) and two mESC lines (D3 and J1). Samples from 492B-4 iPSCs on day 13 were used as a control to normalize data. ( c ) The expression of IM marker genes analysed by RT–PCR is shown. The data from three independent experiments are presented as the means±s.d. ( n =3) in a and b . For mPSCs, we generated EBs without any inducing factors, and then the same two-step treatment was employed as used for hPSCs. Full size image Characterization of developmental potential of human IM cell During mouse development, Osr1 + IM cells contribute to renal, gonadal and adrenocortical cells [18] . After culturing the OSR1 + cells isolated on culture day 11 using the single-cell method for an additional 7 days with 100 ng ml −1 BMP7 and 100 ng ml −1 Wnt3a or 1–3 μM CHIR99021, the expression of marker genes for various IM-derived organs was elevated, including RET , SALL4 and HOXB7 for nephric duct and ureteric bud, SIX2 and HOXD11 for metanephric mesenchyme, FOXD1 for metanephric stroma, AQUAPORIN 1 ( AQP1 ), PODOCALYXIN and E-CADHERIN for the adult kidney, and DAX1 , LHX9 , SF1 , GATA4 , GATA6 and HSD3β2 for gonadal or adrenocortical cells ( Fig. 7a ). We also found cells that were positive for metanephric kidney markers, such as Lotus tetragonobulus lectin (LTL) and AQP1 for proximal renal tubule, peanut agglutinin and PODOCALYXIN for glomerulus, αSMA for smooth muscle, Dolichos biflorus agglutinin (DBA) and SALL4 for ureteric bud, and epithelial markers, CYTOKERATIN and E-CADHERIN ( Fig. 7b and Supplementary Table S1 ). The OSR1 + cells also differentiated into cells that stained positively for gonadal or adrenocortical markers, GATA4, GATA6 and HSD3β ( Fig. 7b ). 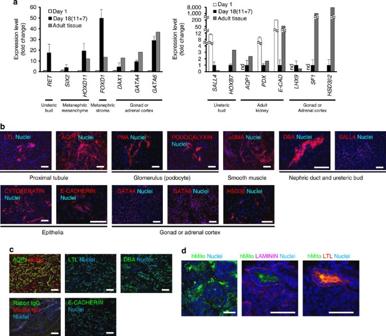Figure 7:In vitroandin vivodifferentiation of OSR1+cells into IM derivatives. (a) The expression of marker genes for the developing kidney, gonad and adrenal cortex in the differentiated cells on culture day 18 (after an additional 7-day culture of the day 11 isolated OSR1+cells differentiated from an OSR1-GFP knock-in hiPSC line, 3D45, using the single-cell method). The mRNAs of human adult kidney were used as controls for the expression ofRET,SALL4,HOXB7,SIX2,HOXD11,FOXD1,AQP1,PODOCALYXINandE-CADHERIN. The mRNAs of human adult testis were used as controls forDAX1andLHX9. The mRNAs of human adult ovary were used as controls forGATA4andGATA6. The mRNAs of human adult adrenal gland were used as controls forSF1andHSD3β2. Each value ofRET,SIX2,HOXD11,FOXD1,DAX1,GATA4andGATA6was normalized to the samples on day 1 before treatments, while that ofSALL4,HOXB7,AQP1,PODOCALYXIN,E-CADHERIN,LHX9,SF1andHSD3β2was normalized to the samples on day 18, whose expression levels in the day 1 samples were so low or much higher than day 18 samples or adult tissues. The data from three independent experiments are presented as the means±s.d. (n=3). nd; not detected. PDX; PODOCALYXIN, E-CAD; E-CADHERIN. (b) The differentiated cells on day 18 were stained with antibodies or lectins against markers for IM derivatives: LTL and AQP1 for proximal renal tubule, peanut agglutinin (PNA) and PODOCALYXIN for glomerular podocytes, αSMA for smooth muscle, DBA and SALL4 for nephric duct and ureteric bud, epithelial markers CYTOKERATIN and E-CADHERIN, and GATA4, GATA6 and HSD3β for the gonads or adrenal cortex. (c) AQP1 and human nuclear antigen (HuNu), control, LTL, E-CADHERIN and DBA staining of histological sections of 4-week-old hiPSC-derived IM grafts transplanted into immunodeficient mice (NOD. CB17-Prkdcscid/J). (d) Immunostaining of the histological sections of organ culture samples collected on day 7 for human mitochondria (hMito) and for LTL or LAMININ. Note that the right two panels are images of the same section. Scale bars, 50 μm. Figure 7: In vitro and in vivo differentiation of OSR1 + cells into IM derivatives. ( a ) The expression of marker genes for the developing kidney, gonad and adrenal cortex in the differentiated cells on culture day 18 (after an additional 7-day culture of the day 11 isolated OSR1 + cells differentiated from an OSR1-GFP knock-in hiPSC line, 3D45, using the single-cell method). The mRNAs of human adult kidney were used as controls for the expression of RET , SALL4 , HOXB7 , SIX2 , HOXD11 , FOXD1 , AQP1 , PODOCALYXIN and E-CADHERIN . The mRNAs of human adult testis were used as controls for DAX1 and LHX9 . The mRNAs of human adult ovary were used as controls for GATA4 and GATA6 . The mRNAs of human adult adrenal gland were used as controls for SF1 and HSD3β2 . Each value of RET , SIX2 , HOXD11 , FOXD1 , DAX1 , GATA4 and GATA6 was normalized to the samples on day 1 before treatments, while that of SALL4 , HOXB7 , AQP1 , PODOCALYXIN , E-CADHERIN , LHX9 , SF1 and HSD3β2 was normalized to the samples on day 18, whose expression levels in the day 1 samples were so low or much higher than day 18 samples or adult tissues. The data from three independent experiments are presented as the means±s.d. ( n =3). nd; not detected. PDX; PODOCALYXIN, E-CAD; E-CADHERIN. ( b ) The differentiated cells on day 18 were stained with antibodies or lectins against markers for IM derivatives: LTL and AQP1 for proximal renal tubule, peanut agglutinin (PNA) and PODOCALYXIN for glomerular podocytes, αSMA for smooth muscle, DBA and SALL4 for nephric duct and ureteric bud, epithelial markers CYTOKERATIN and E-CADHERIN, and GATA4, GATA6 and HSD3β for the gonads or adrenal cortex. ( c ) AQP1 and human nuclear antigen (HuNu), control, LTL, E-CADHERIN and DBA staining of histological sections of 4-week-old hiPSC-derived IM grafts transplanted into immunodeficient mice (NOD. CB17- Prkdc scid /J). ( d ) Immunostaining of the histological sections of organ culture samples collected on day 7 for human mitochondria (hMito) and for LTL or LAMININ. Note that the right two panels are images of the same section. Scale bars, 50 μm. Full size image To assess the developmental potential of hiPSC-derived IM cells in vivo , we transplanted day 11 OSR1 + cells generated with single-cell method into the epididymal fat pads (EFPs) of immunodeficient mice (NOD. CB17- Prkdc scid /J). At 4 weeks after transplantation, grafts from nine independent experiments contained cells immunoreactive for renal markers, such as AQP1, LTL, E-CADHERIN and DBA ( Fig. 7c ) without developing either teratomas or forming lineage cells other than IM derivatives ( Supplementary Fig. S10 ). The ability of hiPSC-derived OSR1 + cells to differentiate into polarized epithelia with tubular structures was examined by coculturing the cells with mouse metanephric cells in organ culture experiments, as described previously [26] . We found that the OSR1 + cells evaluated after treatment with 10 ng ml −1 TGFβ1 for an additional 7 days were integrated into mouse metanephric tissues to form renal structures. Some of the OSR1 + IM-derived cells constituted polarized tubule-like structures, which were positive for both a proximal tubule marker (LTL) and LAMININ, a marker for polarized epithelia ( Fig. 7d ). We examined a total of 354 organ culture samples (162 with hiPSC-derived OSR1 + cells and 192 with control untreated hiPSCs) and found that human LTL + LAMININ + tubule-like structures originated from OSR1 + IM cells in 8 organ culture samples out of 162 (4.94%). On the other hand, when we cocultured untreated hiPSCs with mouse metanephric cells, the human cells did not form kidney-like structures or express any of the markers ( n =192; 0%; P =0.0017). We found only a few human DBA + ureteric bud lineage cells differentiated from hiPSC-derived OSR1 + cells in the organ cultures ( Supplementary Fig. S12 ). These data suggest that IM cells induced from hPSCs using our differentiation protocols can differentiate into IM derivatives in vitro and in vivo , and also indicated that they have the developmental potential to contribute to three-dimensional renal structures. Gene targeting in hPSCs has proven to be technically difficult, and around 20 genes have so far been successfully targeted in hPSCs [27] . The efficient gene targeting in hPSCs has been performed using zinc-finger nucleases [27] , transcription activator-like effector nucleases [28] or adeno-associated viruses [29] , [30] . BAC-based approaches were also used to disrupt both alleles of ATM or p53 by sequential targeting in hESCs [31] . We have herein extended these findings to generate GFP reporter lines in hiPSCs, which can be used for monitoring the differentiation of the cell lines. We have also made use of the combination of Taqman qPCR and SNP array analyses to detect homologous recombinants. The BAC-based strategy has led to the efficient targeting of 3% of drug-resistant clones. As BAC clones contain the entire length of target genes, it was speculated that longer homologous arms from BAC-based vectors might more efficiently induce homologous recombination. Our results indicate the applicability of BAC-mediated strategies to target genes in hPSCs. Several studies conducted on the differentiation of ESCs into IM and kidney lineages have demonstrated the difficulty of isolating and examining the differentiated cells [9] , [10] , [11] , [12] , [13] , [14] , [15] . The generation of reporter lines in this study enables the quantitative monitoring of the IM differentiation from hiPSCs, and also allowed us to examine the gene expression and the developmental potential of purified IM cells. Two-dimensional cultures are simple differentiation formats suitable for studying developmental mechanisms and for screening drug compounds. The reporter lines and induction methods established in this study ( Fig. 8 ) could provide powerful tools for elucidating the mechanisms of IM and kidney lineage commitment. 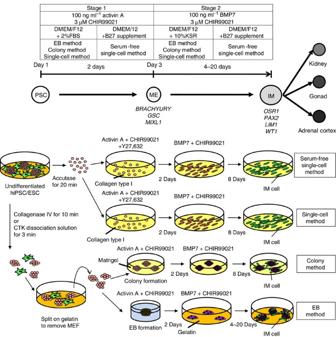Figure 8: Schematic illustrations of two-step differentiation methods from hPSCs through ME into IM cells. Applied factors and media are summarized in boxes. Marker genes that help characterize cells within particular domain are shown below developmental stages. Figure 8: Schematic illustrations of two-step differentiation methods from hPSCs through ME into IM cells. Applied factors and media are summarized in boxes. Marker genes that help characterize cells within particular domain are shown below developmental stages. Full size image The iPSC technology enables the creation of patient-derived hPSC lines and in vitro disease models for studying the pathophysiology and for identifying therapeutic drug compounds. Other clinical applications include the use of iPSC-derived cells for replacement therapy and in vitro toxicology studies [32] . However, the efficiency and frequency of generating the differentiated renal cell types, such as glomerular podocytes and renal tubular cells, or three-dimensional renal structures from hPSC-derived IM cells in this study is low and not sufficient to be used in the development of these strategies. Therefore, the next step in developing new strategies for the treatment of kidney diseases will require subsequent studies to develop both specific and efficient methods to differentiate hPSC-derived IM cells into renal lineage cells, by modifying the induction protocols established in our current study. In addition, the targeted protocols to differentiate IM cells into other IM derivatives, such as adrenal cortex and gonad, should be devised as well for regenerative medicine strategies in the fields of endocrinology and reproductive medicine. Cell culture hiPSCs (201B6, 201B7, 253G1 and 253G4) and hESCs (H9, khES1 and khES3) were grown on feeder layers of mitomycin C-treated mouse embryonic fibroblasts (MEF) derived from embryonic day (E) 12.5 ICR mouse embryos in media containing Primate ES medium (ReproCELL) supplemented with 500 U ml −1 penicillin/streptomycin (Invitrogen) and 4 ng ml −1 recombinant human basic fibroblast growth factor (Wako). For routine passaging, hiPSC colonies were dissociated by an enzymatic method with CTK dissociation solution consisting of 0.25% trypsin (Invitrogen), 0.1% collagenase IV (Invitrogen), 20% KSR (Invitrogen) and 1 mM CaCl 2 in PBS, and split at a ratio between 1:3 and 1:6. BAC recombineering The human BAC clone RP11-458J18, which contains all of the exons of the OSR1 gene and extends from 86.3 kb upstream to 89.8 kb downstream of the gene locus, was purchased from BACPAC Resource Center at the Children’s Hospital, Oakland Research Institute (Oakland, CA). Recombineering was performed as described [33] . Briefly, the BAC clone was introduced into E. coli strain DH10B. To construct the knock-in vector, we designed two primers which have short sequences of the homologous recombination regions of the OSR1 gene with the 5′ or 3′ end of EGFP-pA-PNL sequence, and performed genomic PCR using KOD Plus Neo polymerase (TOYOBO) according to the manufacturer’s protocol. The primers used for genomic PCR were as follows: hOSR1-EGFP-S, 5′-TCTTCTTTTCTTTGCAGATCCGGATTGAGAAGCCACTGCAACTACCGAACACCATGGTGAGCAAGGGCGAGGA-3′; hOSR1-PNL-AS, 5′-GTTCACTGCCTGAAGGAAGGAGTAGTTGGTGAGCTGCAGGGAAGGGTGGAGTCGACGGCGAGCTCAGACG-3′. Then, the targeting vector, EGFP-pA-PNL cassette containing 5′ and 3′ homology arms, was electroporated into DH10B containing BAC RP11-458J18 and activated recombinases. The transformed bacteria were plated on LB plates with appropriate antibiotics and incubated overnight at 37 °C. Selected clones were picked and subjected to PCR to confirm whether the EGFP-pA-PNL cassette was integrated into the OSR1 endogenous locus through successful homologous recombination. Genetic modification of hiPSCs Electroporation was performed as previously described [34] with some modifications. The human OSR1-EGFP-pA-PNL BAC vector was linearized by restriction enzymes and sterilized by ethanol precipitation. hiPSCs (201B7) were treated with 10 μM ROCK inhibitor Y27,632 (Wako) overnight and trypsinized. Cells were then centrifuged and resuspended in PBS. A total of 30 μg of linearized DNAs was added into the resuspended hiPSCs. The cells were subjected to a single 250 V, 500 mF pulse (Gene pulser CE, Bio-Rad) at room temperature and plated on feeder layers of mitomycin C-treated STO cells. Antibiotic selection was applied 2 days after electroporation. Taqman PCR assay Real-time PCR reactions were carried out with 100 ng of genomic DNA, 250 nM of Taqman probes and 500 nM of primers. The sequences of the primers were as follows: OSR1F, 5′-GGATTGAGAAGCCACTGCAACT-3′; OSR1R, 5′-CCGTTCACTGCCTGAAGGA-3′ and OSR1 probe, 5′-(FAM)CAAGGTTTTGCTGCCC(MGB)-3′. Removal of PGK-Neo cassette The hiPSCs with a targeted OSR1 allele were treated with 10 μM Y27,632 overnight and trypsinized. Cells resuspended in PBS were electroporated with 30 μg of pCXW-Cre-Puro as described above and plated on feeder layers of mitomycin C-treated STO cells. Antibiotic selection was applied a week after electroporation. SNP array analysis Genomic DNA was analysed on GeneChip Mapping 250K NSP arrays (Affymetrix) according to the manufacturer’s protocol. The genomic copy numbers, including allele-specific copy numbers (AsCNs), were calculated using the CNAG/AsCNAR software program as previously described [35] . Genetic lesions, including copy number gains and losses, were detected using a hidden Markov model-based algorithm implemented in the CNAG/AsCNAR software program [36] . Differentiation protocols For EB formation from hiPSC/ESCs, a 10-cm plate containing hiPSCs with 80% confluency was rinsed with PBS and treated with 1 mg ml −1 collagenase IV in DMEM for 10 min at 37 °C. The collagenase solution was rinsed away with PBS and replaced with Stage 1 medium containing DMEM/F12+Glutamax (Invitrogen) supplemented with 500 U ml −1 penicillin/streptomycin and 2% FBS (HyClone). The cells were then scraped off with a cell scraper, dissociated by pipetting and distributed into a low attachment six-well plate (NALGENE NUNC) containing Stage 1 medium, 100 ng ml −1 recombinant human/mouse/rat activin A (R&D Systems) and 100 ng ml −1 recombinant mouse Wnt3a (R&D Systems or StemRD) or 1–3 μM CHIR99021 (Wako). To differentiate cells towards the IM, EBs on culture day 3 were transferred onto gelatin-coated plates. The cells were cultured for an additional 20 days with Stage 2 medium containing DMEM/F12+Glutamax supplemented with 0.1 mM non-essential amino acids, 500 U ml −1 penicillin/streptomycin, 0.55 mM 2-mercaptoethanol, 10% KSR, 100 ng ml −1 recombinant human BMP7 (R&D Systems) and 100 ng ml −1 recombinant mouse Wnt3a or 1–3 μM CHIR99021. Before differentiation with the colony method, hiPSC colonies grown on a MEF feeder layer were dissociated by an enzymatic method with CTK dissociation solution, incubated on gelatin-coated plates for 30 min to remove MEFs, and seeded on Matrigel-coated plates (BD) with MEF conditioned Primate ES medium containing 10 ng ml −1 basic fibroblast growth factor. When hiPSC colonies attained ~70% confluency, the same induction method used for the three-dimensional EB method described above was implemented. For the single-cell method, hiPSC/ESC colonies grown on a MEF feeder layer were first dissociated by an enzymatic method with CTK dissociation solution and incubated on gelatin-coated plates for 30 min to remove MEFs. Then, the cells were dissociated to single cells by gentle pipetting after the treatment with Accutase (Innovative Cell Technologies, Inc.) for 20 min and seeded on Human Collagen Type I-coated plates (BD) at a density of 1.5 × 10 5 cells cm −2 . The same inducing factors described above was used, except for the addition of 10 μM Y27,632 to the Stage 1 treatment. For the serum-free single-cell method, the cells were cultured with a serum-free medium containing DMEM/F12+Glutamax supplemented with 1 × B27 supplements (Invitrogen) and 500 U ml −1 penicillin/streptomycin throughout the differentiation culture. For miPSC/ESCs, cells were dissociated with 0.25% trypsin/EDTA and split onto gelatinized plates. After incubation for 30 min to remove feeder cells, EBs were generated by 2-day hanging drop culture from 1,000 undifferentiated iPSCs or ESCs in 20 μl undifferentiation medium without leukaemia inhibitory factor. Then, EBs were plated onto gelatinized 24-well plates (30 EBs per well) and cultured with Stage 1 treatment for 2 days, followed by Stage 2 treatment for additional days, as indicated. Long-term culture of OSR1(GFP) + cells hiPSC-derived OSR1(GFP) + cells on culture day 11 were isolated by flow cytometry sorting, seeded onto gelatin-coated 96-well plates at a density of 1.0 × 10 4 cells per well, and cultured with Stage 2 medium containing 10 μM Y27,632. After overnight incubation, 100 ng ml −1 recombinant human BMP7 and 100 ng ml −1 recombinant mouse Wnt3a or 1–3 μM CHIR99021 were added to the medium, and cells were cultured for an additional 7 days. After the culture, cells were examined by immunostaining. Graft preparation and implantation hiPSC-derived OSR1 + and OSR1 − cells on culture day 11 were isolated by flow cytometry sorting, seeded onto low attachment 96-well plates (NALGENE NUNC) at a density of 1.0 × 10 5 cells per well, and cultured with Stage 2 medium containing 10 μM Y27,632 for 2 days. Then about 20 aggregates were transferred onto polyethylene terephthalate fiber-Collagen Sponge (MedGEL) that was prewetted with Stage 2 medium. The aggregates and Sponge were overlayed with 50 μl of Matrigel. The resultant implant constructs were placed in an incubator set at 37 °C and 5% CO 2 for 1 h to allow the construct to gel. These constructs were transferred to culture dishes with prewarmed medium until implantation. One of the EFPs of immunodeficient mice (NOD. CB17- Prkdc scid /J) was carefully externalized through an abdominal incision, then a single implant construct was wrapped in the EFP and the implanted EFP were returned to abdominal cavity. After 4 weeks of implantation, mice were killed and the serial sections of implanted tissues were examined with immunostaining. Organ culture experiment hiPSC-derived OSR1(GFP) + cells on culture day 11 were isolated by flow cytometry sorting, seeded onto gelatin-coated 24-well plates at a density of 5.0 × 10 4 cells per well, and cultured with Stage 2 medium containing 10 μM Y27,632 and 10 ng ml −1 recombinant human TGFβ1 (R&D Systems) for 7 days. Embryonic day 11.5 metanephric kidneys from ICR mice were dissected in improved MEM (Invitrogen). The metanephric kidneys were then placed in 0.05% trypsin-EDTA for 10 min at 37 °C and dissociated by pipetting. Dissociated cells were stabilized in kidney culture medium containing improved MEM supplemented with 500 U ml −1 penicillin/streptomycin and 10% FBS for 10 min at 37 °C, and then filtered through a 40-μm cell strainer (BD). A total of 10 × 10 4 freshly dissociated metanephric cells and 1 × 10 4 of TGFβ1-treated hiPSC-derived OSR1(GFP) + cells dissociated by Accutase were mixed, seeded onto 96-well low-cell-adhesion plates (Lipidure Coat, NOF) with adding 10 μM Y27,632, then cultured for overnight at 37 °C to form aggregates. The aggregates were cultured at air–fluid interface on 0.4-μm pore polycarbonate filter (Millipore) supplied with kidney culture medium at 37 °C. After 1 week of organ culture, the aggregates were fixed and the serial sections were examined with immunostaining. Stained sections were analysed with an LSN710 confocal microscope (Zeiss). The statistical significance of the difference in frequency of renal tubule formation between hiPSC-derived OSR1 + cells and control undifferentiated hiPSCs in organ culture was analysed using Fisher’s exact test. How to cite this article: Mae, S.-I. et al. Monitoring and robust induction of nephrogenic intermediate mesoderm from human pluripotent stem cells. Nat. Commun. 4:1367 doi: 10.1038/ncomms2378 (2013).